Time-resolved compression of a capsule with a cone to high density for fast-ignition laser fusion The advent of high-intensity lasers enables us to recreate and study the behaviour of matter under the extreme densities and pressures that exist in many astrophysical objects. It may also enable us to develop a power source based on laser-driven nuclear fusion. Achieving such conditions usually requires a target that is highly uniform and spherically symmetric. Here we show that it is possible to generate high densities in a so-called fast-ignition target that consists of a thin shell whose spherical symmetry is interrupted by the inclusion of a metal cone. Using picosecond-time-resolved X-ray radiography, we show that we can achieve areal densities in excess of 300 mg cm −2 with a nanosecond-duration compression pulse—the highest areal density ever reported for a cone-in-shell target. Such densities are high enough to stop MeV electrons, which is necessary for igniting the fuel with a subsequent picosecond pulse focused into the resulting plasma. Over the last four decades, a tremendous effort has been devoted to studying the physics of high-density matter by compressing spherical shells with powerful laser beams [1] , [2] . Achieving high compression with pressures ~10 16 Pa is vital for inertial confinement fusion [3] , where a few milligrams of frozen deuterium (D) and tritium (T) fuel are compressed by laser light ablation (direct drive) or by X-ray ablation (indirect drive) to such high temperatures and densities that ignition is reached and a thermonuclear burn wave spreads throughout the shell. Laboratory compression experiments reach similar pressures that exist inside astrophysical objects, providing an important means for studying those material states [4] , [5] . Pressures of ~10 16 Pa prevail in the sun’s core, whereas they are ~100 × lower in the core of giant planets. An important step towards ignition has been recently demonstrated by measuring fusion energy that exceeds the energy coupled in the fuel in an inertial confinement fusion implosion [6] . So far, ignition has not been reached despite code predictions. Besides the conventional ‘hot-spot’ approach, which triggers ignition in the centre of a rapidly converging shell, alternative approaches such as fast ignition (FI) [7] and shock ignition [8] , which separate the compression and ignition phases of the implosion, have been proposed. Ignition is achieved from highly localized heating: on the side of the high-density fuel using a separate ultrahigh-intensity laser (FI) or in the centre of the compressed shell by a converging shock wave (shock ignition). These concepts are attractive because higher gains might be achievable than with central hot-spot ignition [9] . Early experiments studying the FI concept [10] , [11] reported a coupling efficiency of 15–30% of the short-pulse laser energy into the compressed plasma. Those experiments were limited by several factors, including insufficient drive-laser energy (2.5 kJ), no pulse-shaping capability and a longer drive-laser wavelength (532 nm instead of 351 nm)—unfavourable factors for achieving high compression. In addition, the low number (nine) of overlapping drive beams resulted in a large illumination nonuniformity that affected the symmetry and possibly the hydrodynamic stability of the implosion. Based on our experiments and simulations, we conclude that the FI experiments [10] , [11] were merely qualitative and were not guided by sufficient simulation capability to adequately describe this complicated radiation–hydrodynamic problem. It therefore seems questionable whether sufficient compression was achieved to stop MeV electrons and surprising that such high coupling efficiencies were reported [10] , [11] (efficiencies that could not be reproduced in experiments on OMEGA [12] ). Follow-up experiments at the Institute for Laser Engineering confirm an insufficient compression, being ~10 × lower than was previously estimated, and a much-lower (~1.6%) short-pulse beam energy coupling [13] . The poor performance of the implosions at the Institute for Laser Engineering might be the result of several factors including a high adiabat ( α >~6) in the shell ( α is defined as the ratio of the plasma pressure in the shell to the Fermi pressure of a degenerate electron gas [14] ), an improperly shaped adiabat profile, breakup of the shell because of hydrodynamic instabilities, or a combination of these factors. A low adiabat ( α =~1 to ~2) is a prerequisite for high-target compression and is achieved by shaping the laser pulse in such a way that the inner portion of the shell, which is not ablated, remains on a low α , whereas the laser raises the α in the ablated outer material in order to reduce the growth of hydrodynamic instabilities [15] . Imploding massive shells with a low implosion velocity (≤2 × 10 7 cm s −1 ) and a shaped low- α profile substantiates a viable path for achieving highly compressed cores for FI [16] . In the experiments reported here, plastic shells with an embedded hollow cone made out of high- Z material were imploded with good laser illumination uniformity using the adiabatic shaping technique [15] . 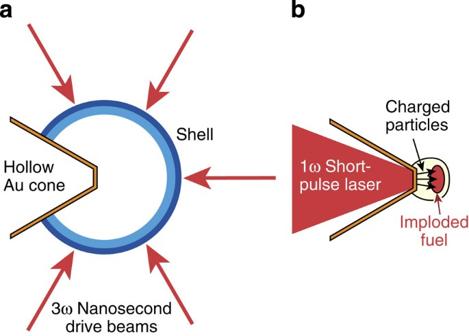Figure 1: Schematic of a direct-drive cone-in-shell experiment. (a) A nanosecond laser implodes a shell consisting of an ablator and a fuel layer around a hollow cone that provides a clear path for a short-pulse laser. (b) The short-pulse laser produces charged particles that ignite the compressed fuel. Figure 1 shows a schematic of a direct-drive cone-in-shell experiment. The purpose of the cone is to provide a plasma-free path for the short-pulse ignition laser to propagate as close as possible to the dense fuel. One complication is that the cone breaks the spherical symmetry and requires multidimensional simulation capability to accurately model both the flow of the material and the interaction between radiation and matter. Figure 1: Schematic of a direct-drive cone-in-shell experiment. ( a ) A nanosecond laser implodes a shell consisting of an ablator and a fuel layer around a hollow cone that provides a clear path for a short-pulse laser. ( b ) The short-pulse laser produces charged particles that ignite the compressed fuel. Full size image Important quantities that characterize the fuel assembly are the mass-density distribution ρ ( r ) and the areal density ρR , which is given by the integral of ρ over the spatial coordinate from the shell’s centre to infinity, Measurements of ρR and ρ provide a method for comparing the actual and predicted implosion performances. ρR and ρ can be obtained experimentally by X-ray radiography [17] . This technique has been used on OMEGA to study the implosion dynamics of deuterium gas-filled plastic shells without a cone using an ~1-ns-laser-driven, ~5-keV broadband backlighter and an X-ray framing camera with an ~40-ps integration time [18] . A mass-density distribution ρ ( r ) and a ρR of up to ~60 mg cm −2 were measured at various times outside of peak compression [18] . Previous experiments with cone-in-shell targets in indirect [19] and direct drive [20] , [21] investigated high-adiabat ( α =6) implosions with simple square pulses, which lacked quantitative comparison to simulations. Here we demonstrate with picosecond, time-resolved radiographic measurements of the hydrodynamic evolution of cone-in-shell implosions that the assembled plasma is dense enough to stop MeV electrons at a time when the cone tip has not been breached by the implosion—an important requirement for FI. This is only possible because of the unique experimental capability of the Omega Laser Facility and a significant improvement in multidimensional simulations. The excellent agreement between experiment and simulation obtained here provides a benchmark for the code calculations that will be used to further improve implosion performance. Experimental setup The current experiment used thicker (42 μm compared with 24 μm) plastic shells with a cone and a lower gas pressure (~0.8 atm of air compared with 15 atm of D 2 gas) imploded by a shaped laser pulse to minimize X-ray self-emission. The previous experiments with the thinner shell and the higher gas pressure were limited by a strong X-ray self-emission from the hot core that prevented a measurement at peak compression [18] . Here a short-pulse laser-driven X-ray source with shorter emission time and a higher photon energy combined with a narrow-bandwidth (Δ E / E =1.2 × 10 −3 ) crystal imager provided the necessary tool to study the fuel assembly in unprecedented detail. The mass-absorption coefficient μ of the compressed material is a function of the photon energy, and measuring it with a spectrally pure photon source significantly decreases the uncertainty in the inference of ρ and ρR . 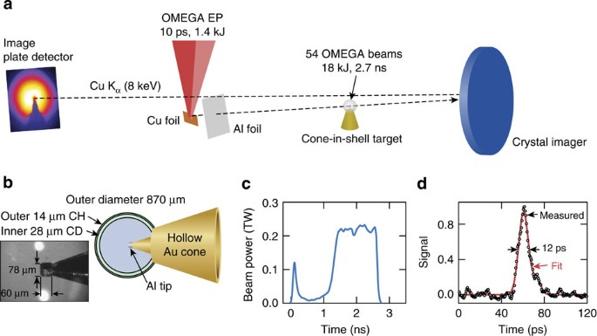Figure 2: Experimental setup. (a) Schematic of the setup of the backlighter experiment with a Cu foil irradiated by the OMEGA EP short-pulse beam and using 54 OMEGA beams to implode a cone-in-shell target. A 50-μm-thick Al foil was located 2 mm from the Cu foil to shield it from plasma and X-ray radiation from the implosion. A raw image of the fuel assembly is shown in the image plane. The distances are not to scale. (b) Illustration of the cone-in-shell target. (c) Laser pulse shape to implode the capsule. (d) Time-resolvedKαX-ray emission from a Cu foil target irradiated with an ~1-kJ, 10-ps pulse. Figure 2a shows the experimental setup. The cone-in-shell target ( Fig. 2b ) consisted of a hollow gold cone mounted inside a plastic shell. A small aluminium cylindrical tip was mounted on the end of the cone. The purpose of the 60-μm thick Al tip was to delay the shock breakout compared with a previous design with a 15-μm Au tip [12] . There is a trade-off between possessing sufficient tip material to delay the breakout and a good electron coupling into the core because more material might affect the electron transport and increases the standoff distance from source to core. The new design does not worsen the electron transport (see Discussion). After imploding the shell with 54 OMEGA ultraviolet beams [1] with an energy of ~18 kJ and the drive pulse shown in Fig. 2c , the infrared (1053, nm wavelength), ~1.4-kJ, 10-ps OMEGA EP short-pulse laser [22] irradiated a thin Cu foil. The OMEGA EP laser was defocused to an ~200-μm spot that provided an intensity of ~5 × 10 17 W cm −2 and generated fast electrons with a kinetic energy in the range of several 100 keV to ~MeV (ref. 23 ). Strong electrostatic sheath fields at the target boundary retain most of the fast electrons in the ~1-mm foil. The electrons recirculate and generate K α radiation, providing a relatively uniform Cu K α area backlighter source. A spherical Bragg crystal imager [24] tuned to the Cu K α1 line (8.048 keV) was located on the opposite side of the target and imaged the implosion onto an image plate detector with a magnification of 14.7. The imaging system efficiently rejects unwanted background and X-ray self-emission from the implosion. The technique also benefits from a higher probing photon energy because the plasma self-emission scales with exp( −hν/kT ), where hν is the photon energy and kT is the plasma temperature. In shots without a backlighter, the background at 8 keV caused by self-emission from the implosion was measured to be ~40 × weaker than the signal of the K α backlighter. Another important parameter for this technique is the emission time of the backlighter, which determines the time resolution, because a time-integrating detector was used. Figure 2d shows a time-resolved measurement of the K α flash [23] by coupling an ultrafast X-ray streak camera to the Bragg crystal imager. A K α emission time of 12 ps was quantified, which is short enough to prevent any spatial blurring from the hydrodynamic motion. Figure 2: Experimental setup. ( a ) Schematic of the setup of the backlighter experiment with a Cu foil irradiated by the OMEGA EP short-pulse beam and using 54 OMEGA beams to implode a cone-in-shell target. A 50-μm-thick Al foil was located 2 mm from the Cu foil to shield it from plasma and X-ray radiation from the implosion. A raw image of the fuel assembly is shown in the image plane. The distances are not to scale. ( b ) Illustration of the cone-in-shell target. ( c ) Laser pulse shape to implode the capsule. ( d ) Time-resolved K α X-ray emission from a Cu foil target irradiated with an ~1-kJ, 10-ps pulse. Full size image Radiographic images First, an image of an undriven target was taken (see Fig. 3a ), where the Al tip is clearly visible and less opaque than the gold cone. This shot provided an independent measurement of the magnification of 14.8±0.1 and a measure of the spatial resolution of 22±3 μm. The backlighter was then used to image imploded targets. The time delay between the implosion laser and short-pulse laser was varied on a shot-to-shot basis to probe the fuel assembly at various times (see Fig. 4a–e ). The false colour scheme represents the measured optical depth given by ln( I 0 /I), where I is the measured transmitted signal and I 0 is the measured backlighter intensity. The frame in Fig. 4a shows the implosion at 3.75 ns after the start of the drive pulse. Time zero is defined as the time when 2% of the peak power from the drive laser pulse is reached. The fuel starts to assemble in front of the tip and the Al tip is compressed to a higher density, which can be seen when comparing the measured optical depth in the Al tip to that of the undriven target. At later times, the Al tip was more deformed and eventually completely destroyed as the fuel assembly reached higher density. Peak compression was reached at the time of the frame in Fig. 4d at T peak =4.05 ns, whereas the last frame was recorded after peak compression at 4.15 ns. Figure 4f–j displays calculated backlighter images for those shots. 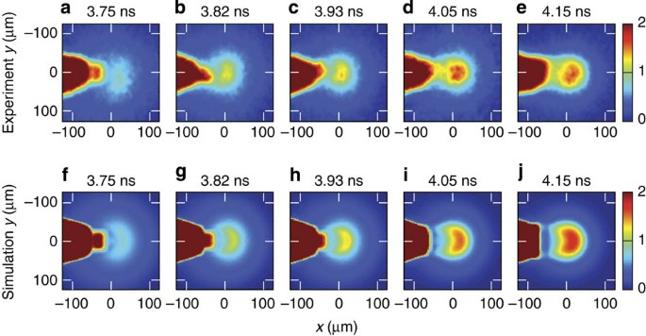Figure 4: Radiographic images of implosion. (a–e) Measured images of cone-in-shell targets at various stages of the implosion. The probing time was measuredin situwith ±0.05-ns accuracy at full energy by operating the neutron temporal diagnostic38in hard X-ray mode. The probing time is with respect to the start of the ultraviolet drive-laser pulse. (f–j) Simulated radiographs from 2D radiation–hydrodynamic simulations. The false colour scheme indicates the optical depth. The simulations were performed with the two-dimensional (2D) radiation–hydrodynamic code DRACO [25] in cylindrical geometry and were post-processed with the code Spect3D [26] . The simulation capability was significantly improved compared with the results reported in ref. 12 . 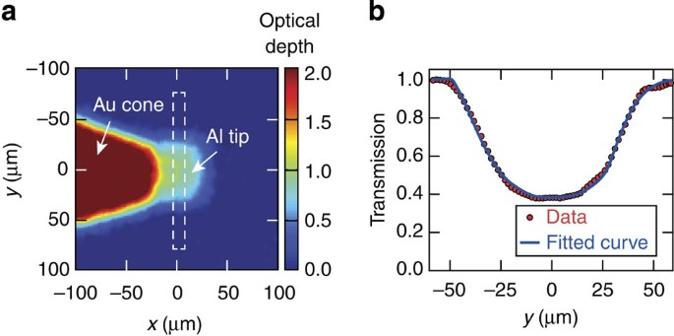The radiation transport has been included, the Eulerian scheme improved, and nonlocal thermal electron transport [27] and cross-beam energy transfer [28] accounted for. Figure 3: Radiograph of undriven target. (a) Flash radiography image of an undriven cone-in-shell target and (b) vertical lineout through the centre of the Al tip calculated from the area marked by the dashed rectangle. The measured transmission is well fitted using the 8.048-keV X-ray transmission through a cold aluminium disk. Figure 3: Radiograph of undriven target. ( a ) Flash radiography image of an undriven cone-in-shell target and ( b ) vertical lineout through the centre of the Al tip calculated from the area marked by the dashed rectangle. The measured transmission is well fitted using the 8.048-keV X-ray transmission through a cold aluminium disk. Full size image Figure 4: Radiographic images of implosion. ( a – e ) Measured images of cone-in-shell targets at various stages of the implosion. The probing time was measured in situ with ±0.05-ns accuracy at full energy by operating the neutron temporal diagnostic [38] in hard X-ray mode. The probing time is with respect to the start of the ultraviolet drive-laser pulse. ( f – j ) Simulated radiographs from 2D radiation–hydrodynamic simulations. The false colour scheme indicates the optical depth. Full size image Shock breakout The breakout time of the shock driven through the cone tip was measured independently, similar to experiments that were described in detail in refs 12 , 21 . The shots were performed by firing only the OMEGA beams and switching off the OMEGA EP beam. The compressing shell pushed a jet of plasma material towards the cone tip and created a shock wave through the cone wall. When the shock wave reached the inner cone surface, it generated optical emission, which was measured temporally and spatially resolved. The measured average breakout time from three implosions was T shock =3.85±0.04 ns, which agrees well with the predicted value of 3.84 ns. Density profiles We inferred the time-resolved radial density distributions and time-resolved areal densities from the measured optical-depth distributions under the assumption of cylindrical symmetry of the plasma along the cone axis. Vertical lineout profiles of the optical depth τ ( y ) (see Fig. 5 ) taken through the dense core show maximum values of up to 1.65 and a full-width at half-maximum as small as ~80 μm. Experimental and simulated ρ ( r ) are compared in Fig. 6a–e at various times. The ρ ( r ) profiles match for radii larger than 50 μm but show slight differences in the dense region. 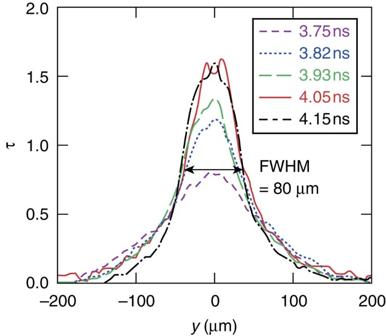Figure 5: Optical-depth profiles. Time-resolved optical-depth lineouts through the dense core of compressed plastic measured at a photon energy of 8.048 keV. Profiles are taken perpendicular to the cone axis. FWHM, full-width at half-maximum. Figure 5: Optical-depth profiles. Time-resolved optical-depth lineouts through the dense core of compressed plastic measured at a photon energy of 8.048 keV. Profiles are taken perpendicular to the cone axis. FWHM, full-width at half-maximum. 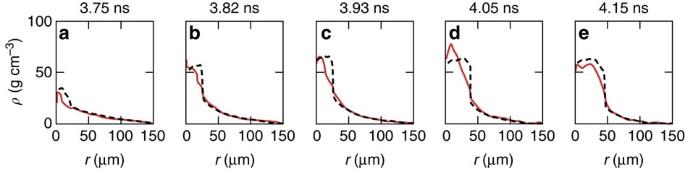Figure 6: Density profiles. Measured (solid) and simulated (dashed) density profiles perpendicular to the cone axis for various times (a–e). Full size image Figure 6: Density profiles. Measured (solid) and simulated (dashed) density profiles perpendicular to the cone axis for various times ( a – e ). Full size image Areal density The inferred ρ ( r ) is integrated to obtain ρR , which is compared with the predicted value ( Fig. 7 ). The measured areal densities agree with the simulations to better than 15%. The laser compressed the plasma to high areal density (~300 mg cm −2 ) at a distance of ~50 μm in front of the cone tip. 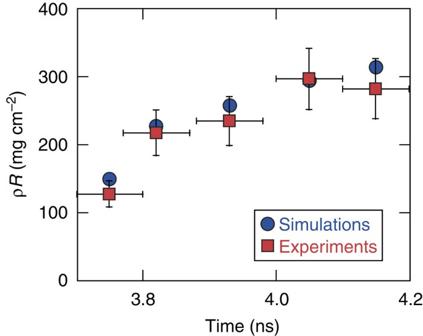Figure 7: Areal density. Measured (squares) and simulated (dots) areal density perpendicular to the cone axis for various times.ρRis determined from the core centre to infinity. Error bars in time are based on the measurement accuracy of the timing diagnostics38. TheρRerror bars are based on a 14% uncertainty in the inferredρR, which is determined from the errors in the measured optical depthτ(12%) and the mass absorption coefficientμ(7%). Theτ-error includes contributions from uncertainties in background subtraction, photon statistics and the reconstruction of the 2-D backlighter intensity distribution. Theμ-error is inferred based on an estimated 10% temperature uncertainty. Figure 7: Areal density. Measured (squares) and simulated (dots) areal density perpendicular to the cone axis for various times. ρR is determined from the core centre to infinity. Error bars in time are based on the measurement accuracy of the timing diagnostics [38] . The ρR error bars are based on a 14% uncertainty in the inferred ρR , which is determined from the errors in the measured optical depth τ (12%) and the mass absorption coefficient μ (7%). The τ -error includes contributions from uncertainties in background subtraction, photon statistics and the reconstruction of the 2-D backlighter intensity distribution. The μ -error is inferred based on an estimated 10% temperature uncertainty. Full size image The simulations compare well with the measured radiographic images, revealing similar structure and size of the imploded plastic material. The simulated optical densities agree to better than 10% with the measured optical densities. Slight differences are observed in the shape of the high-density region, which might be caused by three-dimensional effects that were not taken into account in the simulations. For late times, some differences are observed in the region between the destroyed Al tip and the dense plasma core (see Fig. 4 ). Although the simulations show a distinctive gap, the gap is less pronounced in the measurements, which could be a result of turbulent plasma behaviour and mixing of ablated Al material with the plastic. No significant mixing of Al and plastic material is noticed in the 2D simulations but could be stronger in reality. Slight shot-to-shot differences in the Al-tip deformation do not affect the overall performance of the implosion. The present target is more resilient against the strong shock from the implosion than a previous design with a gold-only cone [12] . Those experiments measured the breakout time for various gold-cone tips with thicknesses from 5 to 15 μm and demonstrated a later breakout for thicker tips. For a 15-μm thickness, the breakout time was 3.76 ns. Therefore, the target with the 60-μm-thick Al tip improved the margin for the arrival of the short-pulse laser by ~90 ps, bringing the ρR at 3.85 ns to ~200 mg cm −2 ( Fig. 7 ), which is ~70% of the peak ρR . The Al-tip target does not worsen the transport of fast electrons through the tip as the areal density of the 60-μm Al+2-μm Au tip is 20 mg cm −2 , whereas the areal density of the 15-μm-thick Au tip is 29 mg cm −2 . The continuous-slowing-down-approximation ranges of fast electrons in Al and Au are comparable: 555 mg cm −2 and 776 mg cm −2 (ref. 29 ) for 1-MeV electrons, respectively. Slightly less areal density is required in Al to completely stop a 1-MeV electron. The 20 mg cm −2 in the Al tip hardly affects the energy loss of a 1-MeV electron and similarly in the 15-μm-thick Au tip. On the other hand, the angular scattering increases with the atomic number of the material and the mean free path for 90° scattering is much shorter in Au (46 mg cm −2 ) than in Al (151 mg cm −2 ) [30] . As scattering increases the divergence of the electron beam when it passes through the tip, the amount of electrons that intercept the dense plasma (the electrons that are available for ignition) decreases. The Al tip might therefore have some advantage compared with the Au-tip design. A simple expression for maximum ρR was derived in ref. 31 for an imploded DT capsule filled with 1 atm of DT gas, which makes it possible for the maximum ρR to be scaled with the drive laser energy E L , the laser wavelength λ and the adiabat α inn of the inner portion of the shell . For the current experiment, E L =18 kJ, λ =0.35 μm and α inn =3.4, for which the simple expression yields ~350 mg cm −2 , only ~17% higher than the actual value, showing that the scaling model can be used to estimate the expected ( ρR ) max for different energies and adiabats. For a laser energy of 1.9 MJ, which was used in a recent experiment [6] at the National Ignition Facility, and for α inn =3.4, a value of ( ρR ) max =1,600 mg cm −2 is estimated, which is a factor of ~4.6 higher than with OMEGA. A higher areal density allows for particle stopping up to a higher kinetic energy and, given a certain distribution of kinetic energies, relaxes the requirement to ignite the fuel. Our simulations indicate that an even higher ρR might be achievable on OMEGA by removing the air from the shell and reducing the power of the laser pulse picket. 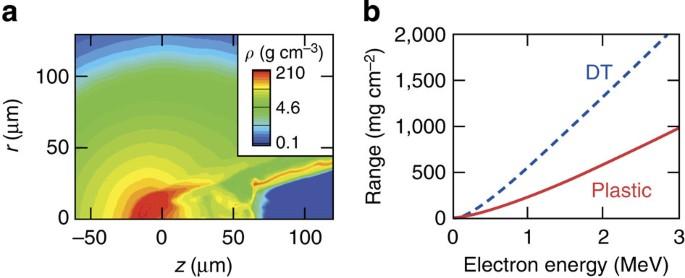Figure 8: Density map and electron stopping. (a) Simulated mass-density distribution of the improved implosion at the time of shock breakout at 3.96 ns, which provides an areal density of 500 mg cm−2. (b) Calculated range of fast electrons in compressed deuterated plastic and DT. Figure 8a shows the calculated mass-density map at shock breakout for the improved design. The mass and energy of the hot spot are decreased, which delays the breakout of the cone tip by reducing the pressure on the cone tip. Fuel stagnation is closer to the target centre with a higher density and higher areal density. It brings the shock breakout as close as 80 ps to the peak compression time. The ablation velocity is only 8% less for the reduced-power picket implosion. In general, a larger ablation velocity improves the hydrodynamic stability [15] , but those implosions use thick shells and a low implosion velocity so the slight reduction in ablation velocity does not significantly affect hydrodynamic stability. The main effect of the reduced picket is a lower α inn and reduced mass and temperature in the hot spot. At the time of shock breakout, the areal density reaches 500 mg cm −2 , 83% of ρR max =600 mg cm −2 . It is important to note that such high areal densities provide sufficiently dense plasma to stop fast electrons. Figure 8b shows the calculated average range of fast electrons in compressed deuterated plastic (solid curve) including blooming and straggling [30] . Electrons up to 1.8 MeV will completely range out in a ρR =500-mg cm −2 plastic plasma, whereas a 200-mg cm −2 plasma stops electrons up to 0.9 MeV. The areal density across the dense core is about twice that value (2 ρR ) for electrons propagating from the centre of the cone tip to the centre of the dense core. Therefore, electrons of up to 1.5 MeV can be stopped along this trajectory for the present implosion and up to 3 MeV for the optimized implosion. The dashed curve in Fig. 8b represents the fast-electron range in compressed DT, which is about twice that of plastic. DT plasma with 550 mg cm −2 will stop a 1-MeV electron. Similar areal densities are expected for imploded cryogenic DT shells on OMEGA. In fact, ρR =300 mg cm −2 has been measured on OMEGA in spherical cryogenic DT implosions (without a cone) [32] . National Ignition Facility implosions with cryogenic DT compressed to 1,600 mg cm −2 will stop electrons up to 2.4 MeV propagating from outside to the plasma centre and up to 4.5-MeV electrons across the dense core. Figure 8: Density map and electron stopping. ( a ) Simulated mass-density distribution of the improved implosion at the time of shock breakout at 3.96 ns, which provides an areal density of 500 mg cm −2 . ( b ) Calculated range of fast electrons in compressed deuterated plastic and DT. Full size image Injecting a short-pulse laser into the hollow cone produces fast electrons with energies of up to several MeV [12] . The coupling efficiency of the electron energy into the dense core depends on a number of parameters, including the standoff distance between the location where the fast electrons are produced and the dense plasma, the divergence and energy distribution of the electrons, the transport dynamics through a potential pre-plasma inside the cone [12] and through the cone wall, and the areal density of the compressed plasma. There is an ongoing effort to quantify this coupling efficiency in OMEGA experiments by characterizing the spatial distribution of fast-electron energy in the compressed core using Cu-doped plastic shells and imaging the fast-electron–excited Cu K α fluorescence emission [33] , [34] . Cone-in-shell target A hollow gold cone with an inner full opening angle of 34°±1°, a sidewall thickness of 15 μm and a small inner 40-μm circular flat tip was inserted into a 42-μm-thick plastic shell with a 14-μm outer CH layer, a 28-μm inner strong deuterated plastic layer and an outer diameter of ~870 μm. The shell was filled with ~0.8 atm of air at shot time. A thin (~2-μm) gold layer inside the cone end served as a mounting layer for the Al tip. The Al tip was 60 μm thick on axis and 78 μm in diameter. Backlighting of undriven target Figure 3a shows a backlighter image of an undriven target. The Al tip was well centred on the Au cone within ±5 μm. The image was corrected for spatially varying backlighter intensity, similar to that described in ref. 18 , and for hard X-rays that were generated in the foil and scattered in the diagnostic. The expected 8-keV X-ray transmission through the Au cone wall is ~7 × 10 −6 , and the area shadowed by the cone should be free of X-ray signal. The high-energy X-ray background that appeared in this area was therefore subtracted from the measured image before the 2D backlighter intensity distribution was reconstructed. The image was then normalized to the backlighter intensity distribution, resulting in the image shown in Fig. 3a . A vertical lineout through the centre of the cylindrical Al tip is well fitted by a convolution of the radial transmission function through a disk, with a Gaussian curve, representing the spatial resolution of the imaging system (see Fig. 3b ). Here κ is the absorption coefficient, r is the disk radius and y is the coordinate of observation. The radius of the Al tip was r =39 μm and the absorption coefficient of cold aluminum at 8.048 keV was κ =1.265 × 10 −2 μm −1 . The fit yielded an independent measurement of the magnification of 14.8±0.1, which is in excellent agreement with the magnification of 14.7 calculated from engineering drawings. A spatial resolution of 22±3 μm was inferred from the fit, which is a factor of ~2 worse than the resolution of ~10 μm reported in ref. 24 . The reason is that the resolution tests in ref. 24 were done with an aperture in front of the crystal, which mitigates the astigmatism of the spherical crystal and improves the spatial resolution, whereas in the current experiment no aperture was used to maximize the signal. Absorption coefficient and mass-absorption coefficient The optical depth τ is given by the integral over the absorption coefficient κ along the path of an X-ray photon through the dense plasma measured at the specific backlighter photon energy. The measured optical-depth profiles τ ( y ) were Abel inverted to infer the absorption coefficient using an iterative Abel algorithm [35] . The assumption of a straight-line photon path is justified at high photon energies. The absorption coefficient is equal to the product of the mass-absorption coefficient μ and the mass density ρ , where μ is a function of plasma electron temperature T e and ρ . A steady-state nonlocal thermal electron calculation of the mass-absorption coefficient μ was performed with the SPECT3D software [26] for C 1 D 1.4 plasma at a photon energy of 8.048 keV and the density profile was inferred ( ρ = κ/μ ). In the range of densities and temperatures of interest here, μ varies between ~3.3 and ~2 cm 2 g −1 along the path of integration, as shown in Fig. 9a . Profiles of ρ and T e from DRACO simulations along the same y direction were used to calculate μ versus position. The technique is sensitive to the assumed temperature and density. A lower temperature results in a higher μ and therefore in a lower inferred ρ . The sensitivity of ρ on the temperature was studied by multiplying the temperature profile from the hydrodynamic simulation by 0.9 and 1.1 and repeating the data analysis. The resulting inferred curves ρ ( r ) are very similar (<±3% deviation) for r >20 μm and deviate slightly more (<±12% deviation) at the centre of the compressed target. The sensitivity of μ on the density is less important and is minimized by an iterative procedure. The inferred density profile is reiterated and μ is recalculated. The process quickly converges. 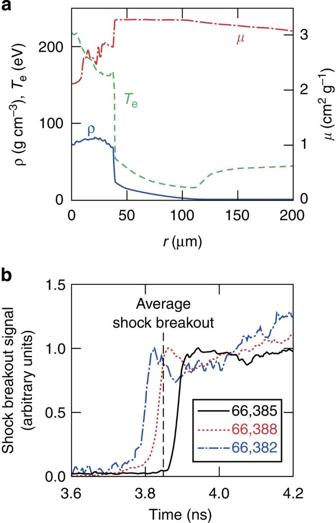Figure 9: Mass-absorption coefficient and shock breakout. (a) NLTE calculation of the radial profile of the mass-absorption coefficient (μ; dashed–dotted curve) of a C1D1.4plasma at a photon energy of 8.048 keV along the photon path through the dense plasma at peak compression (4.05 ns) using density (solid) and temperature (dashed) profiles from the radiation hydrodynamic simulation. (b) Shock breakout measured with a streaked optical pyrometer for three different implosions. The average shock breakout time is marked by the vertical dashed line. Figure 9: Mass-absorption coefficient and shock breakout. ( a ) NLTE calculation of the radial profile of the mass-absorption coefficient ( μ ; dashed–dotted curve) of a C 1 D 1.4 plasma at a photon energy of 8.048 keV along the photon path through the dense plasma at peak compression (4.05 ns) using density (solid) and temperature (dashed) profiles from the radiation hydrodynamic simulation. ( b ) Shock breakout measured with a streaked optical pyrometer for three different implosions. The average shock breakout time is marked by the vertical dashed line. Full size image Shock breakout measurements The abrupt onset of optical emission was measured temporally and spatially resolved from the inside of the cone with a streaked optical pyrometer (SOP) [36] in the ~600- to 750-nm-wavelength range and with two velocity interferometer systems for any reflector (VISARs) [37] at a 532-nm wavelength. Figure 9b shows the SOP signal for three different implosions. Slight differences in pulse shape and shell thickness give rise to the variation in breakout time. The SOP integrates over a time period of 150 ps, determined by the slit width and the sweep speed of the streak camera. The signal is differentiated with respect to time and the first peak determines shock breakout with an accuracy of ±40 ps. The VISAR achieves a higher accuracy of ±20 ps in measuring shock breakout with the help of a faster streak camera. For each shot, the measurements of all three instruments are in agreement within the experimental error. How to cite this article: Theobald, W. et al . Time-resolved compression of a capsule with a cone to high density for fast-ignition laser fusion. Nat. Commun. 5:5785 doi: 10.1038/ncomms6785 (2014).